In vitroproduction of fertile sperm from murine spermatogonial stem cell lines Spermatogonial stem cells (SSCs) are the only stem cells in the body that transmit genetic information to the next generation. The long-term propagation of rodent SSCs is now possible in vitro , and their genetic modification is feasible. However, their differentiation into sperm is possible only under in vivo conditions. Here we show a new in vitro system that can induce full spermatogenesis from SSC lines or any isolated SSCs. The method depends on an organ culture system onto which SSCs are transplanted. The settled SSCs form colonies and differentiate up into sperm. The resultant haploid cells are fertile, and give rise to healthy offspring through micro-insemination. In addition, the system can induce spermatogenesis from SSCs that show spermatogenic failure due to a micro-environmental defect in their original testes. Thus, an in vitro system is established that can be used to correct or manipulate the micro-environmental conditions required for proper spermatogenesis from murine SSC lines. The maintenance of mammalian spermatogenesis depends on the presence of spermatogonial stem cells (SSCs). The self-renewing proliferation of SSCs and their differentiating division, followed by the sequential proliferation of daughter spermatogonia, are required to support spermatogenesis [1] . The differentiated spermatogonia undergo meiotic recombination and reductive cell division to form haploid cells. The round haploid spermatids then change their shape dynamically into sperm [2] . The duration of this process from SSCs to sperm takes 35 and 64 days in mice and humans, respectively [3] . The process is not germ cell-autonomous, but requires orchestrated support from the micro-environmental milieu produced by surrounding somatic cells, especially Sertoli and Leydig cells [4] , [5] . Trials to achieve spermatogenesis in vitro , have faced many difficulties and remained incomplete [6] , [7] . On the other hand, the in vitro proliferation of murine SSCs has become possible by adding glial cell line-derived neurotrophic factor to the SSCs culture media [8] , [9] . The cultured SSCs, termed germline stem (GS) cells or SSC lines, proliferated in a self-renewing manner for up to or beyond 2 years, while remaining stable genetically, epigenetically and karyotypically [10] . It has been reported that genetic modifications were feasible in GS cells [11] , [12] . Nonetheless, it has not yet been possible to induce spermatogenesis from these cells in vitro . To produce sperm from GS cells, we had to resort to systems using in vivo conditions such as cell transplantation in the seminiferous tubules [13] , or a method using the reconstructive nature of immature testicular cells [14] . These in vivo methods are useful for certain purposes, such as to test the functional properties of SSCs. However, because they are not free from complex influences from the host body, they offer only a slight advantage over the original testicular spermatogenesis method when trying to elucidate the mechanism or nature of spermatogenesis. Therefore, an in vitro system for spermatogenesis has been desired for the study of spermatogenesis. Very recently, we developed an organ culture system that supported the complete spermatogenesis of mice from primitive spermatogonia up to sperm [15] . In the present study, we combined this organ culture method with existing technologies: GS cell culturing and cell transplantation into the seminiferous tubules of host testis, to develop an in vitro system of spermatogenesis, which encompasses the proliferation of SSCs, their homing to niches, and differentiation into sperm ( Supplementary Fig. S1 ). This in vitro system induced spermatogenesis even from SSCs and a GS cell line originally showing spermatogenic failure owing to a defect in the testicular micro-environment. Thus, we successfully produced an in vitro system for the induction of complete spermatogenesis from murine GS cells. Colonization of injected GS cells in cultured tissues In in vivo transplantation experiments, SSCs introduced into the seminiferous tubules migrate from the lumen towards the periphery of the tubule and settle on the basement membrane. After settling, SSCs begin proliferation along the basement membrane to form colonies. When the size reaches several millimeters in length along the tubule, the differentiation of germ cells commences at the centre of each colony [16] . These phenomena observed in transplantation experiments could be viewed as the homing of SSCs into their niches, followed by their proliferation and differentiation [17] . To examine whether such a homing phenomenon of SSCs also takes place in vitro , we injected green fluorescent protein-expressing GS cells (GFP-GS cells), derived from pCXN-GFP [18] transgenic mice, into the testes of W/W v pup mice (2.5–8.5 days postpartum (dpp)), which contain very few germ cells because of genetic defects of the c-kit gene. Tissue fragments of the host testes were cultured on an agarose gel according to the organ culture method [15] , [19] ( Fig. 1a ). The GFP-GS cells in the seminiferous tubules remained in the lumen for several days, but signs of migration towards the periphery of the seminiferous tubules were observed as early as 2 h after transplantation ( Fig. 1b ). At 12 h, some cells were already present on the basement membrane. Until day 3, most GS cells resided on the basement membrane. They also appeared to have started proliferation at around day 7 or earlier. On day 14, basal compartments of some seminiferous tubules were occupied by GS cells ( Fig. 1c ). We observed the cultured tissues for more than a week, which revealed that GFP-GS cells were increasing in number ( Fig. 1d ). In addition, cell division of GS cells was documented based on the presence of phospho-histon-H3 (PHH3)-positive GS cells at both 9 and 18 days after transplantation [20] ( Fig. 1e ). Together, these findings indicate that GS cells can form colonies in the seminiferous tubules even under culture conditions that lack active circulatory systems. 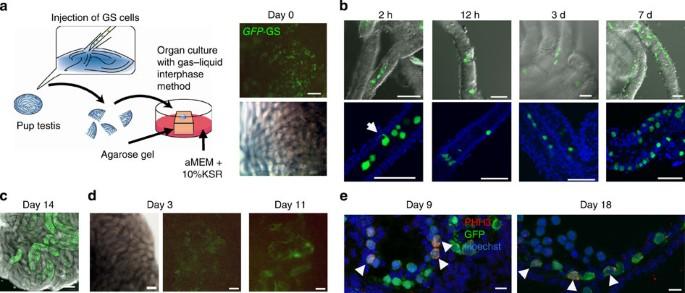Figure 1: Scheme of experiment and behaviour of transplanted GS cells in the cultured testis tissue fragments. (a) GFP-GS cells were injected into the seminiferous tubules of pup mouse testes at 2.5–8.5 dpp. The tissue fragments of host testes were placed on agarose gel half-soaked in the medium. The GS cells spread and floated in the lumen of seminiferous tubules directly after transplantation. (b) The behaviour of GS cells was tracked by observing whole-mount pictures captured with confocal laser microscopy (CLM) at 2 h, 12 h, 3 days, and 7 days. The upper row shows differential interface contrast images merged with GFP, whereas the lower row shows immunostaining pictures with antibody to GFP (green) and Hoechst staining (blue). Arrow indicates a pseudopod formation, a sign of migration. (c) Image of CLM on day 14. (d) Fixed-point observation through days 3–11. (e) Immunostaining of cryosections (on days 9 and 18) of host testis fragments with antibodies to PHH3 (red) and GFP (green), counterstained by Hoechst (blue). Several GS cells were dividing (arrowheads) judged by PHH3-positive. Scale bars: 200 μm (a,c,d); 50 μm (b); 10 μm (e). Figure 1: Scheme of experiment and behaviour of transplanted GS cells in the cultured testis tissue fragments. ( a ) GFP-GS cells were injected into the seminiferous tubules of pup mouse testes at 2.5–8.5 dpp. The tissue fragments of host testes were placed on agarose gel half-soaked in the medium. The GS cells spread and floated in the lumen of seminiferous tubules directly after transplantation. ( b ) The behaviour of GS cells was tracked by observing whole-mount pictures captured with confocal laser microscopy (CLM) at 2 h, 12 h, 3 days, and 7 days. The upper row shows differential interface contrast images merged with GFP, whereas the lower row shows immunostaining pictures with antibody to GFP (green) and Hoechst staining (blue). Arrow indicates a pseudopod formation, a sign of migration. ( c ) Image of CLM on day 14. ( d ) Fixed-point observation through days 3–11. ( e ) Immunostaining of cryosections (on days 9 and 18) of host testis fragments with antibodies to PHH3 (red) and GFP (green), counterstained by Hoechst (blue). Several GS cells were dividing (arrowheads) judged by PHH3-positive. Scale bars: 200 μm ( a , c , d ); 50 μm ( b ); 10 μm ( e ). Full size image Spermatogenesis from GS cells in cultured tissues To confirm that GS cells are able to proceed up to or beyond the meiotic phase of spermatogenesis, we exploited 2 lines of transgenic mice, Acr-GFP [21] , [22] and Gsg2-GFP [23] , to establish GS cells from them. We confirmed that the GS cells derived from Acr-GFP ( Acr -GS cells) and Gsg2-GFP ( Gsg2 -GS cells) expressed GFP at the expected phases of differentiation, mid- and end-meiotic, respectively, when transplanted in the testis in vivo (data not shown). Host testes of wild-type mice were pretreated with busulfan once, in the prenatal period from 12.5–15.5 days postcoitum (dpc) [24] , to deplete endogenous germ cells. When the host testes fragments injected with Acr -GS cells were cultured, GFP expression was observed from days 18–30. The expression lasted for 16–45 days ( Fig. 2a,c ). Testis tissues receiving Gsg2 -GS cells, on the other hand, showed GFP expression from days 22–41 and lasted for 14–38 days in culture ( Fig. 2b,c ). Meiosis in mouse testes starts at around 7 dpp (ref. 25 ), and the Acr -GFP in the transgenic mice begins expression at around 15 dpp (ref. 21 ). The delays in GFP expression in the injected Acr -GS cells might reflect the time required for settling and proliferation before meiosis starts. In the case of Gsg2 -GS cells, the same is suggested. As for the frequency of GFP expression, it was observed in 44 of 49 testes injected with Acr -GS cells (89.8%) and in 14 of 15 testes injected with Gsg2 -GS cells (93.3%) ( Table 1 ). These data strongly suggest that in vitro meiosis from GS cells took place in the explanted testis tissues. To confirm that the meiosis was genuine, we employed an immunohistochemical technique using an antibody for synaptonemal complex protein 1 (SYCP1) [7] , a specific marker of meiosis, and another for GFP. The SYCP1-antibody demonstrated a spread of chromosomes typical of meiosis in spermatocytes, while the GFP-antibody revealed an acrosomal dot in spermatids when Acr -GS cells were incubated in the explants ( Fig. 2d–f ). Regular histological sections with Periodic acid-Schiff (PAS) staining also showed an acrosomal cap structure on the nuclei of round spermatids in the W/W v host testes ( Fig. 2g ). In addition, we used an antibody to mouse sperm protein 56 (SP56) [26] , a sperm-specific protein that localizes to the sperm surface and in the acrosomal matrix, and found many positive cells in the centre of seminiferous tubules ( Supplementary Fig. S2 ). Liberated spermatids, both round and elongating, and sperm were observed when cultured tissues were mechanically dissociated ( Fig. 2h–j ). 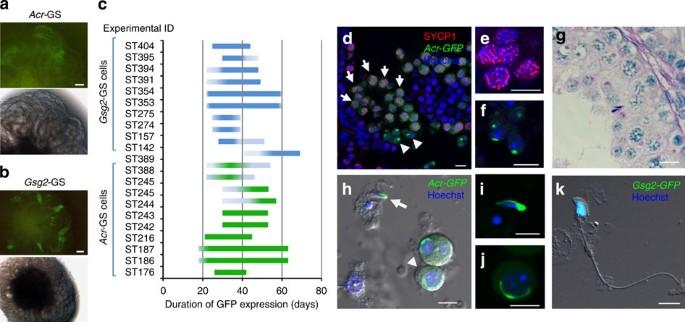Figure 2: Spermatogenesis from GS cellsin vitro. (a) A testis tissue fragment transplanted withAcr-GS cells showed GFP expression from culture day 23. (b) A testis tissue fragment transplanted withGsg2-GS cells showed GFP expression from culture day 21. (c) Periods of GFP expression derived fromAcr- andGsg2-GS cells cultured in pup mouse testis fragments from busulfan-treated wild-type orW/Wvmice. Horizontal bar indicates corresponding age of the host mice. (d) Immunostaining of host testis tissue cryosections, transplanted withAcr-GS cells cultured for 40 days. Anti-SYCP1 (red), anti-GFP (green), and counterstain with Hoechst 33342 dye (blue) were merged. Many double-positive cells (arrows) and cells with an acrosomal cap (arrowheads) were observed. (e) A magnified view of cells in meiosis stained with anti-SYCP1 and Hoechst 33342 dye. (f) A magnified view of haploid cells stained with anti-GFP and Hoechst 33342 dye. (g) PAS staining of culturedW/Wvtestis receiving transplantation ofGsg2-GS cells. Spermatocytes and round and elongating spermatids were identified. (h) Cells were dissociated from the cultured testis tissues on day 53. The transplantedAcr-GS cells developed into round (step 8; arrowhead) and elongating (step 12; arrow) spermatids. (i) A magnified view of an elongating spermatid. (j) Another example of a round spermatid. (k)Gsg2-GS cells transplanted into host testis matured into sperm during 57 days of organ culture. A confocal image merged with GFP and Hoechst (blue). Scale bars: 200 μm (a,b); 10 μm (d–k). The frequencies of haploid cell formation, judged by any one method of histological, immunohistochemical, or acrosomal GFP identification, were 31.3 and 40.0% among GFP-positive tissues injected with Acr - and Gsg2 -GS cells, respectively ( Table 2 ). The flagellated sperm were observed in 3 of 17 GFP-expressing samples examined after mechanical dissociation ( Fig. 2k ). The number of sperm found was more than 10 in each tissue. Flow cytometric analyses of cultured testis tissues, either of busulfan-treated wild-type or W/W v mice, injected with Acr -GS cells were performed using 6 tissue fragments in each experiment. Among the whole dissociated cells, Acr-GFP -expressing cells, that is, meiotic cells, comprised 0.41 and 0.27% of the total in busulfan treated-wild type or W/W v mice, respectively ( Supplementary Fig. S3 ). These Acr -GFP-positive cells, 777 and 641 in number, included 3 and 14 round spermatids identified by having GFP-positive acrosomes, respectively. One sperm was identified in the latter. Together, these findings indicate that GS cells differentiated into spermatids occasionally, and into sperm in some cases, in the explanted host testis tissues. Figure 2: Spermatogenesis from GS cells in vitro . ( a ) A testis tissue fragment transplanted with Acr -GS cells showed GFP expression from culture day 23. ( b ) A testis tissue fragment transplanted with Gsg2 -GS cells showed GFP expression from culture day 21. ( c ) Periods of GFP expression derived from Acr - and Gsg2 -GS cells cultured in pup mouse testis fragments from busulfan-treated wild-type or W/W v mice. Horizontal bar indicates corresponding age of the host mice. ( d ) Immunostaining of host testis tissue cryosections, transplanted with Acr -GS cells cultured for 40 days. Anti-SYCP1 (red), anti-GFP (green), and counterstain with Hoechst 33342 dye (blue) were merged. Many double-positive cells (arrows) and cells with an acrosomal cap (arrowheads) were observed. ( e ) A magnified view of cells in meiosis stained with anti-SYCP1 and Hoechst 33342 dye. ( f ) A magnified view of haploid cells stained with anti-GFP and Hoechst 33342 dye. ( g ) PAS staining of cultured W/W v testis receiving transplantation of Gsg2 -GS cells. Spermatocytes and round and elongating spermatids were identified. ( h ) Cells were dissociated from the cultured testis tissues on day 53. The transplanted Acr -GS cells developed into round (step 8; arrowhead) and elongating (step 12; arrow) spermatids. ( i ) A magnified view of an elongating spermatid. ( j ) Another example of a round spermatid. ( k ) Gsg2 -GS cells transplanted into host testis matured into sperm during 57 days of organ culture. A confocal image merged with GFP and Hoechst (blue). Scale bars: 200 μm ( a , b ); 10 μm ( d – k ). Full size image Table 1 Comparison of GFP expression frequency in testis tissues transplanted with Acr -GS and Gsg2 -GS cells. BUS, busulphan. Full size table Table 2 The frequency of haploids in testis tissues injected with three GS cells. Full size table Fertility of haploids derived in vitro from GS cells Finally, we tested the fertility of haploid cells derived from GS cells in vitro by micro-insemination. Acr -GS or GFP-GS cells were injected into the testes receiving prenatal busulfan treatment on 13.5 dpc, which were then cultured as explants for 43 days. The explants were dissociated to collect round spermatids, which were used to micro-inseminate 68 oocytes employing the ROSI technique [27] . Five offspring were delivered and grew healthily ( Fig. 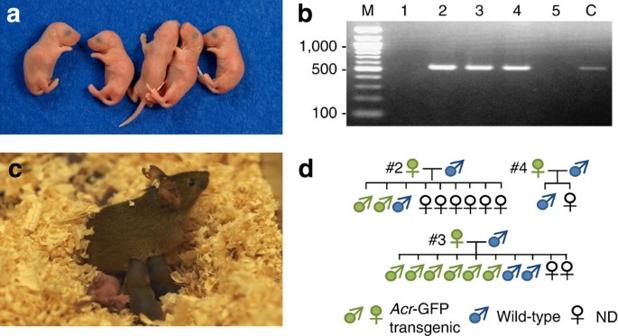Figure 3: Offspring from GS cell-derived gametes. (a) Offspring were produced using round spermatids derived fromAcr-GS cellsin vitroemploying the ROSI technique. (b) Tail tip DNA was subjected to PCR analysis for GFP. Three pups were positive for GFP. M: marker (ladders of 100 bp); 1–5: pups produced; C: positive control. (c) The offspring delivered an F2 generation following natural mating. (d) Pedigrees of 3 GFP-positive pups. 3a Table 3 ). Three of the five pups carried the GFP gene, indicating their origin to be from Acr -GS cells ( Fig. 3b ). As Acr -GS cells were heterogeneous for the transgene, the pups negative for GFP were either from Acr -GS cells or endogenous germ cells of host testes. The offspring were all female and 3 GFP-positives were mated with wild-type males (ICR) to test their reproductive potential. All became pregnant and delivered 21 pups in total ( Fig. 3c, d ). Eight out of the twelve males of this second generation carried the Acr-GFP gene, which was confirmed by GFP expression in their testes ( Fig. 3d ). It is noteworthy that the Acr -GS cells were derived from 8-day-old pup mice and cryopreserved for 2 years and 9 months. The cells were cultured for 26 days before transplantation into the tissue explants for in vitro spermatogenesis. We also performed ROSI with round spermatids derived from Gsg2 -GS cells cultured in testis tissues of W/W v mice, which produced two offspring, one male and one female ( Table 3 ). The Gsg2 -GS cells were derived from a 4-week-old mouse, and propagated in culture for 24 weeks, with 13 subculturings and 6 weeks of cryopreservation, before being subjected to in vitro spermatogenesis. Figure 3: Offspring from GS cell-derived gametes. ( a ) Offspring were produced using round spermatids derived from Acr -GS cells in vitro employing the ROSI technique. ( b ) Tail tip DNA was subjected to PCR analysis for GFP. Three pups were positive for GFP. M: marker (ladders of 100 bp); 1–5: pups produced; C: positive control. ( c ) The offspring delivered an F2 generation following natural mating. ( d ) Pedigrees of 3 GFP-positive pups. Full size image Table 3 Summary of ROSI data. Full size table Effect of host testes manipulation on in vitro colonization of GS cells In in vivo experiments, it is necessary to deplete endogenous germ cells of host testes or use mutants lacking germ cells for the successful colonization of donor germ cells [13] . Although the presence of endogenous germ cells does not necessarily abolish donor cell colonization in the case of neonatal recipients, it is still desirable to deplete them by pre-treatment [28] . In fact, in our in vitro spermatogenesis system, the expression frequency of GFP derived from Acr -GS cells was lower with host testes of non-treated wild-type mice than that of busulfan-treated or W/W v mice ( Table 1 ). To identify whether this lower frequency of spermatogenesis occurrence might result from a lower colonization efficiency, we used GFP-GS cells to monitor their colonization extent in three groups of host testes: non-treated wild-type, busulfan-treated, and W/W v mice. GFP-GS cells were injected into the testes of each group, aged 2.5–8.5 dpp, followed by the culturing of tissue fragments. Colonization areas of GFP-GS cells in each cultured testis fragment, as a percentage of the total area observed from above with a stereomicroscope, were on average 6.4, 40, and 46% in non-treated, busulfan-treated, and W/W v mouse testes groups, respectively ( Supplementary Fig. S4 , Supplementary Table S1 ). These data indicate that the depletion of endogenous germ cells was favourable for donor germ cell colonization in vitro as well as in vivo . To make the experimental system fully in vitro , we tried to exclude in vivo transplantation procedures from the experimental scheme. Thus, we removed testes from mice that had been pretreated with busulfan at 14.5 dpc, and preserved them for 4–20 h at 4 °C. GFP-GS cells were then injected into the seminiferous tubules of each testis ( Supplementary Fig. S1b ). The transplanted GS cells showed a similar extent of colonization as presented above during tissue culture ( Supplementary Fig. S5a ). When Acr -GS cells were transplanted into the preserved testes, GFP expression started from 17 days in cultured tissue fragments ( Supplementary Fig. S5b ). These results show that testes removed from the body and preserved for at least a few hours can act as hosts to accommodate SSCs and support spermatogenesis. Mature testes as hosts for in vitro spermatogenesis As described above and in our previous report [15] , immature testis tissues can support the full spermatogenesis of both indigenous and transplanted germ cells in vitro . If testes of adult animals are useful as host tissues, the system would become more widely applicable. Therefore, we tested mature testes of 3-week-old W/W v mice as host tissue for GS cells. The transplanted Gsg2 -GS cells expressed GFP from 48 days of culture onward and differentiated into round spermatids ( Fig. 4a–c ). This indicates that not only immature testes but also mature adult testes could be useful as host tissues to support spermatogenesis from GS cells. 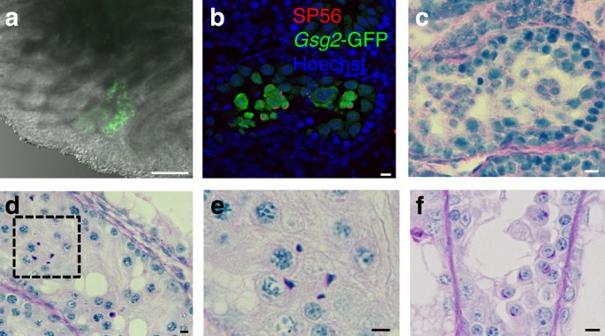Figure 4: Mature testes as the host tissue andin vitrospermatogenesis from SSCs ofSl/Sldmice. (a)Gsg2-GS cells were transplanted into the testes of 3-week-oldW/Wvmice. The fragments of host testes were explanted, and GFP expression detected from day 27. (b) The tissues were cryosectioned and stained with anti-SP56 (red) and anti-GFP (green), and counterstained with Hoechst (blue). (c) The cryosections were stained with the PAS reaction, which showed acrosomes of round spermatids. (d) Cells ofSl/Sldmouse testes were transplanted into explanted testes ofW/Wvmice, 5.5 dpp. Tissues cultured for 50 days were prepared for PAS staining. Areas in rectangles are enlarged in (e). (e) Elongated spermatids were observed. (f)Sl/Sldmouse-derived GS cells were transplanted into explanted testes ofW/Wvmice, 8.5 dpp. Tissues cultured for 52 days were prepared for PAS staining. Acrosomal caps of round spermatids were observed. Scale bars: 200 μm (a); 10 μm (b–f). Figure 4: Mature testes as the host tissue and in vitro spermatogenesis from SSCs of Sl/Sl d mice. ( a ) Gsg2 -GS cells were transplanted into the testes of 3-week-old W/W v mice. The fragments of host testes were explanted, and GFP expression detected from day 27. ( b ) The tissues were cryosectioned and stained with anti-SP56 (red) and anti-GFP (green), and counterstained with Hoechst (blue). ( c ) The cryosections were stained with the PAS reaction, which showed acrosomes of round spermatids. ( d ) Cells of Sl/Sl d mouse testes were transplanted into explanted testes of W/W v mice, 5.5 dpp. Tissues cultured for 50 days were prepared for PAS staining. Areas in rectangles are enlarged in ( e ). ( e ) Elongated spermatids were observed. ( f ) Sl/Sl d mouse-derived GS cells were transplanted into explanted testes of W/W v mice, 8.5 dpp. Tissues cultured for 52 days were prepared for PAS staining. Acrosomal caps of round spermatids were observed. Scale bars: 200 μm ( a ); 10 μm ( b – f ). Full size image Induction of spermatogenesis from SSCs of Sl/Sl d mice in vitro Lastly, we exploited this system to rescue spermatogenic failure due to micro-environmental defects of testes. As a model of such a condition, Sl/Sl d mice were used, which show no spermatogenesis due to the loss of stem cell factor on the surface of Sertoli cells [29] . We dissociated testis cells of Sl/Sl d mice and transplanted them into the testes of W/W v mice and cultured their fragments. Fifty days later, we observed spermatogenesis up to elongating spermatids in histological sections of the explants ( Fig. 4d,e ). In addition, we established GS cells from Sl/Sl d mice, being propagated for 2 months, and introduced them into explants of W/W v mouse testes. In this case, spermatogenesis was observed up to round spermatids ( Fig. 4f ). The round spermatids were observed in 3 out of 9 samples examined in histological sections stained with PAS-hematoxylin ( Table 2 ). In this study, we demonstrated that GS cells can produce fertile spermatids and sperm in vitro by combining a cell transplantation technique and organ culture method ( Supplementary Fig. S1 ). GS cells transplanted in testes, which were then separated into small pieces and cultured on agarose, migrated towards the basal membrane and settled on it, as in the in vivo process. The efficiency of this homing of GS cells appeared surprisingly high and almost comparable to that in vivo . Furthermore, the settled GS cells started proliferation over the basement membrane to form colonies, which was also the same as in vivo . The GS cells then began to differentiate to form sperm in the cultured testis tissues. A new discovery in the present study is the homing and colonization process of GS cells, which were promising signs of successful sperm production in vitro , because the differentiation of SSCs on the basement membrane was already demonstrated in our previous study [15] . The mechanism of SSC migration from the lumen to the basal compartment of the seminiferous tubule is not fully understood [17] . The organ culture system would be useful to elucidate SSCs' behaviour, including homing and colonization, in the seminiferous tubules. Our present study could be interpreted to have transformed a classic experiment of spermatogonial transplantation that uses host animals as a whole into a new in vitro experiment using only testes of host animals. The difference in manipulation of the two experiments would become much more significant when larger animals are used as hosts in the future. In this sense, we reasoned that it would be favourable if the testes were surgically removed beforehand from the host animals and preserved for a while before the injection of SSCs. The experiments on GS cell injection into the preserved mouse testes demonstrated that such an experimental scheme would be feasible. In addition, we demonstrated that not only neonatal testes but also adult testes could be used as a source of host testis tissues. This versatility in the manipulation and source of host testis tissues are encouraging data that promise the wider application of the technique in the future. There have been three strategies reported to be effective for treating spermatogenic defects of Sl/Sl d mice. In the first method, SSCs of Sl/Sl d mice were transplanted into recipients, such as W/W v mice, that can provide normal testicular conditions. The SSCs showed complete spermatogenesis, and the fertility of resultant sperm was demonstrated [30] . In the second method, defective Sertoli cells of Sl/Sl d mice were partially replaced by transplantation of normal Sertoli cells from wild-type mice [31] . This method is theoretically attractive but the efficiency of Sertoli cell transplantation is low, which is a technical hurdle of this method. The third method used a gene-therapy strategy to introduce the Steel gene into the defective Sertoli cells of Sl/Sl d mice by adeno- or lenti-viral transductions [32] , [33] . This method also proved effective to produce fertile sperm in the testes of Sl/Sl d mice. Our present method is based on the same concept as the first method, and made it more feasible and applicable by transforming the system into one that is entirely in vitro . Although this strategy does not seem directly applicable in a clinical situation, it certainly presents a platform for the development of new therapeutic and diagnostic modalities in the future. In conclusion, it is noteworthy that the present system could be used to produce sperm from any cells that have a spermatogenic potential. In this regard, germ cells or primordial germ cells reported or claimed to have been derived from ES/iPS cells and epiblast cells [34] , [35] , [36] , [37] could be tested regarding their spermatogenic activity with our in vitro system. This particular application of our method would break the boundary between germ and somatic cells, and open a new phase in germ cell research. Animals Three lines of transgenic mice, pCXN-GFP [18] , Gsg2/Haspin - GFP [23] , and Acr - GFP [21] , [22] , were used to produce GS cells. The pCXN-GFP mice were provided by Dr. Okabe, Gsg2/Haspin - GFP mice were provided by Dr. Tanaka, and Acr - GFP mice were provided by RIKEN BRC through the National Bio-Resource Project of MEXT, Japan. They were maintained by mating with ICR or C57BL/6 (CLEA Japan). ICR and WBB6F1- W/W v (Japan SLC) were used to prepare host testes for explants. For prenatal busulfan treatment, pregnant ICR mice received an intra-peritoneal single injection of busulfan (40 mg kg −1 ) during 12.5–15.5 dpc (ref. 24 ). WBB6F1- Sl/Sl d mice (Japan SLC) were used as a source of donor SSCs or GS cells. Mice were housed in air-conditioned rooms, 24±1 °C and 55±5%, with 14 h-light and 10 h-dark lightning cycle. The Gsg2/Haspin-GFP mice were housed in a conventional room, while the other mice were kept in a specific pathogen free room. The MF hard pellets (Oriental Yeast) were fed ad libitum . Drinking water was acidified to pH 2.8–3.0 by HCl. All animal experiments conformed to the Guide for the Care and Use of Laboratory Animals and were approved by the Institutional Committee of Laboratory Animal Experimentation (Animal Research Center of Yokohama City University, Yokohama, Japan). Culture of GS cells To establish GFP-GS cells, male pCXN-GFP transgenic mice were mated with wild-type ICR females to produce F1 pups. The testes of F1 pups were dissected and used as a source of GS cells. As the pCXN-GFP transgenic mice express GFP in every cell type, including germ cells, the established GFP-GS cells also expressed GFP. As for Acr - and Gsg2 -GS cells, pup testes of Acr - GFP, Gsg2 - GFP transgenic mice (genetic background was a mixture of ICR, C57Bl/6 and DBA2) were used. GS cells were also established from WBB6F1- Sl/Sl d mice, at 6-weeks-old. For the derivation of GS cells [8] , testis cells were dissociated enzymatically with 2 mg ml −1 of collagenase digestion (Type IV) for 15 min, followed by 1 mM EDTA and 0.25% trypsin for 10 min at 37 °C (ref. 38 ). The singly dissociated cells were incubated overnight in dishes caoted with 0.2% (w/v) gelatin to remove fibroblasts that adhere to the base. The cells were collected by brisk pipetting, and were plated into another well. After 1–3 passages, when fibroblast proliferation diminished, the cells were plated in wells with mouse embryonic fibroblast feeder cells. These feeder cells were pretreated with mitomycin C and placed in a well coated with 0.2% (w/v) gelatin. The culture medium consisted of StemPro-34 SFM (Invitrogen) supplemented with StemPro supplement (Invitrogen), 25 μg ml −1 insulin, 100 μg ml −1 transferrin, 60 μM putrescine, 30 nM sodium selenite, 6 mg ml −1 D-(+)-glucose, 30 μg ml −1 pyruvic acid, 1 μl ml −1 dl-lactic acid (Sigma-Aldrich), 5 mg ml −1 bovine serum albumin, 2 mM L -glutamine, 5×10 −5 M 2-mercaptoethanol, minimal essential medium (MEM) vitamin solution (Invitrogen), MEM non-essential amino acid solution (Invitrogen), 10 −4 M ascorbic acid, 10 μg ml −1 d-biotin (Sigma-Aldrich), 20 ng ml −1 recombinant human epidermal growth factor (Wako pure chemical industries), 10 ng ml −1 human basic fibroblast growth factor (Becton Dickinson), 10 ng ml −1 recombinant human glial cell line-derived neurotrophic factor (R&D Systems), and 1% fetal bovine serum, ES cell-qualified (Invitrogen). The cells were maintained at 37 °C in an atmosphere of 5% carbon dioxide in air. Culture medium was changed every 2–4 days. Cell passage was arbitrary depending on the proliferation state of GS cells in each well. Injection and organ culture method Donor GS cells were collected with 0.25% trypsin digestion for 10 min, and resuspended in the GS cell culture medium at about 10–100×10 6 cells per ml. Donor testicular cells were isolated from the testes of WBB6F1- Sl/Sl d mice, at 5.5 dpp, using same enzymes described above for GS cell derivation. After passing through a cell strainer with a 40-μm pore size (Becton Dickinson, #352340), the cells were suspended in GS cell culture medium, at about 2–10×10 6 cells ml −1 . These single-cell suspensions were injected into the seminiferous tubules through rete testis [38] . The testes that received GS cell transplantation were immediately removed. Otherwise, the testes were removed from the body and then received GS cell injection. In either case, the testes were decapsulated and gently separated by forceps into 1–8 pieces of 2–3 mm in diameter. The tissue fragments were then positioned on stands made of 1.5% agarose gel placed in culture plate wells. Each gel was loaded with 1–3 testis tissue fragments. The amount of medium was adjusted so that it would come up to half-to-four-fifths of the height of the agarose gel. Medium change was performed once a week. The culture incubator was supplied with 5% carbon dioxide in air and maintained at 34 °C. The culture medium used for organ culture was α-Minimum essential medium (α-MEM) (Invitrogen: 12000-022), supplemented with 10% KnockOut serum replacement (Invitrogen: 10828-028). Observations and immunohistochemistry The cultured tissues were observed every 3–7 days under a stereomicroscope equipped with an excitation light for GFP (Olympus SZX12; Olympus) to record the GFP expression of the tissues. For histological examination, the specimens were fixed with Bouin's fixative and embedded in paraffin. One section showing the largest cut surface was made for each specimen and stained with PAS. For immunofluorescence staining, tissues fixed with 4% paraformaldehyde in PBS were cryo-embedded in OCT compound (Sakura Finetechnical) and cut into 7-μm-thick sections. For whole-mount immunohistochemistry, cultured testis tissues were soaked in PBS and seminiferous tubules were untangled with fine tungsten needles. They were fixed with 4% paraformaldehyde in PBS for 30 min and then were treated with methanol for 30 min. Incubation with first antibodies was performed overnight at 4 °C, followed by rinsing twice, and then second antibodies were applied for 1 h at room temperature. Nuclei were counterstained with Hoechst 33342 dye. Specimens were observed with a microscope (Nikon Eclipse TE200) or confocal laser microscope (Olympus FV-1000D). For the observation of spermatids and sperm, cultured tissues were mechanically dissociated using needles to release cells into the PBS. The cell suspension was stained with Hoechst 33342 dye and observed with a microscope under GFP excitation light. The following antibodies were used as the primary antibody: rabbit anti-PHH3 antibody (1:100; Upstate Biotechnology), rabbit anti-SYCP1 antibody (1:600; Novus Biologicals), mouse anti-mouse sperm protein SP56 antibody (1:100; QED Bioscience), rat anti-GFP antibody (1:1000, Nacalai Tesque), and rabbit anti-GFP Alexa Fluor 488 conjugate (1:50; Invitrogen). The secondary antibodies used were goat anti-mouse IgG, goat anti-rabbit IgG, and goat anti-rat IgG, conjugated to Alexa 488 or Alexa 555 (1:200; Molecular Probes). Flow cytometric analysis The cultured testis tissue fragments were treated with 2 mg ml −1 of collagenase for 15 min, followed by 0.25% trypsin and 1 mM EDTA digestion for 10 min at 37 °C to dissociate cells. After passing through a cell strainer with a 40-μm pore size (Becton Dickinson), the cells were suspended in PBS containing 3% fetal bovine serum and subjected to flow cytometry to analyse and sort GFP-expressing cells using a Moflo sorter (Dakocytomation). Micro-insemination The cultured testes tissues were dissected under a stereomicroscope. Round spermatids were collected and injected into the ooplasm of mature wild-type B6D2F1 oocytes using a Piezo-driven micro-manipulator. After full condensation of the spermatid chromosomes, oocytes were then activated by treatment with SrCl 2 in the presence of cytochalasin B to resume meiosis while preventing the extrusion of the segregated female and male chromosomes as polar bodies. After the formation of two female pronuclei, one was removed with a micro-pipette [27] . The fertilized oocytes were cultured for 24 h, and two-cell embryos were transferred into the oviducts of pseudopregnant ICR females. Live fetuses retrieved on Day 19.5 were raised by lactating ICR foster mothers. PCR analysis Genomic DNA was extracted from the mouse tail with a DNeasy Tissue kit (QIAGEN). The DNA samples (10 ng) were added to a 20-μl reaction mixture containing 0.25 μM of each enhanced green fluorescent protein (EGFP) -specific primer and Premix Ex Taq (Takara Bio). EGFP-specific primers were 5′-TACGGCAAGCTGACCCTGAA-3′ and 5′-TGTGATCGCGCTTCTCGTTG-3′. The reaction profile was: 30 cycles of denaturation at 95 °C for 60 s, annealing at 60 °C for 30 s, and extension at 72 °C for 60 s. How to cite this article: Sato, T. et al . In vitro production of fertile sperm from murine spermatogonial stem cell lines. Nat. Commun. 2:472 doi: 10.1038/ncomms1478 (2011).